Reply to: Failure to apply standard limit-of-detection or limit-of-quantitation criteria to specialized pro-resolving mediator analysis incorrectly characterizes their presence in biological samples 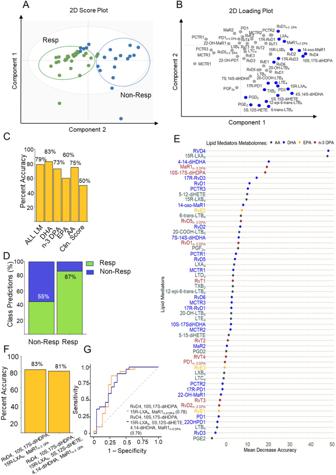Fig. 1: Reanalysis of baseline plasma lipid mediator profiles supports their potential utility as biomarkers. Plasma was collected from RA patients prior to the initiation of treatment with DMARDs and lipid mediator concentrations established using LC-MS/MS-based lipid mediator profiling (seeSupplementary Methodsfor details).A,BOPLS-DA analysis of peripheral blood lipid mediator concentrations for DMARD responders (Resp) and DMARD non-Responders (Non-Resp).ATwo-dimensional score plot with the gray circle representing the 95% confidence regions.BTwo-dimensional loading plots. Lipid mediators with VIP score greater than 1 are highlighted in blue and upregulated in Non-Resp. Results are representative ofn= 30 Resp andn= 22 Non-Resp.CPercentage accuracy score of prediction models based on the combination of all lipid mediators identified and quantified (AL LM) or individual fatty acid metabolomes as indicated. Clin. Score = clinical score (see methods from Gomez et al., for parameters included).DClassification predictions for each class (sensitivity and specificity) of the n-3 DPA model. Green indicates the samples that were predicted as Resp while blue indicates those patients predicted Non-Resp. Percentages indicate true positives (Resp class) and true negatives (Non-Resp class).ERelevance of lipid mediators in the prediction performance of the “ALL LM” model based on decreasing accuracy.FPercentage accuracy score of models using the indicated SPM.GReceiver operating characteristic (ROC) curves and AUC values for predictive models based on the indicated SPM. All the models were created using the random forest methodology (“randomForest” package from R). Data acquisition, multivariate analysis and machine learning models were performed as detailed in Gomez et al. [1] . For the calculation of s/n ratios the AutoPeak and Noise filtering, and Relative Noise functions in SCIEX OS v2.1 were employed. See Supplementary Methods . Reporting summary Further information on research design is available in the Nature Portfolio Reporting Summary linked to this article.